Interlocked loops trigger lineage specification and stable fates in theDrosophilanervous system Multipotent precursors are plastic cells that generate different, stable fates at the correct number, place and time, to allow tissue and organ formation. While fate determinants are known to trigger specific transcriptional programs, the molecular pathway driving the progression from multipotent precursors towards stable and specific identities remains poorly understood. Here we demonstrate that, in Drosophila neural precursors, the glial determinant glial cell missing (Gcm) acts as a ‘time bomb’ and triggers its own degradation once the glial programme is stably activated. This requires a sequence of transcriptional and posttranscriptional loops, whereby a Gcm target first affects the expression and then acetylation of the fate determinant, thus controlling Gcm levels and stability over time. Defective homeostasis between the loops alters the neuron:glia ratio and freezes cells in an intermediate glial/neuronal phenotype. In sum, we identify an efficient strategy triggering cell identity, a process altered in pathological conditions such as cancer. Lineage specification, the process that restricts the potential of multipotent precursors, involves the implementation of a novel transcriptional programme, however, many determinants are only expressed transiently, begging questions as to the molecular pathway ensuring stable identity and terminal differentiation. To understand how this is achieved in vivo , we used a simple model. The Drosophila central nervous system develops from stem cell-like precursors called neuroblasts (NBs) that produce neurons and glia [1] . The glide/gcm gene (glial cell deficient/glial cell missing, referred to as gcm ) codes for a transiently expressed transcription factor that is necessary and sufficient for the differentiation of all lateral embryonic glia. Lack of Gcm transforms most lateral glia into neurons, whereas its forced expression converts neural precursors into glia [2] , [3] , [4] , [5] . Thus, Gcm provides an ideal tool to analyse the pathway underlying lineage specification. gcm activates several targets that implement the glial fate [6] , [7] , [8] including Repo (reversed polarity), a homeodomain transcription factor permanently expressed in all lateral glia [9] , [10] , [11] . Interestingly, Gcm and Repo boost their own expression on autoregulation [4] , [12] and transiently coexist [2] , [3] , [9] , [10] , [13] , [14] . Thus, we hypothesized that Repo acts as a molecular relay, regulating the threshold and dynamic accumulation of Gcm that is necessary for gliogenesis. We show that Drosophila Creb binding protein (dCBP), a histone acetyltransferase (HAT) [15] regulates Gcm stability. dCBP interacts with and triggers the acetylation of Repo and Gcm, which also interact with each other and the three factors are shared components of two interlocked loops. On the one hand, Repo positively regulates gcm gene expression and dCBP induces Gcm stability, on lysine acetylation. On the other hand, Repo induces Gcm degradation in a dosage-dependent manner and dCBP enhances Repo-mediated Gcm degradation. Thus, dCBP and Repo positively regulate Gcm transcriptionally at the beginning of the gliogenic pathway, when Repo starts being expressed, and negatively regulate it posttranscriptionally at a later stage, when Repo accumulates at high levels. The intimate link between the trigger and the consolidator of the glial fate ensures the proper neuron:glia ratio and a stable glial identity. Breaking the homeostasis alters the ratio and freezes cells in a neuronal–glial intermediate state. In sum, this work identifies the molecular network controlling glial specification and the mode of action of the fate determinant. Gcm and Repo positively control gcm expression Cell specification is a binary decision, a type of process that often relies on threshold levels of signalling molecules. We thus dissected the quantitative control of the glial determinant and its impact on the process. Gcm has a dosage-dependent gliogenic effect [16] ( Fig. 1a,b top panels) and positively autoregulates [4] , [12] (see the induction of endogenous transcripts on Gcm ectopic expression in the neurogenic region, scabrous-gal4 (sca) driver; Fig. 1c ). Moreover, autoregulation depends on Gcm levels ( Fig. 1a,b ), as seen by following β-galactosidase (βgal) labelling in embryos expressing increasing gcm doses in a gcm rA87 line, which expresses the lacZ gene under the control of the gcm promoter [4] , [12] ( Supplementary Fig. 1a ). Finally, using a strong gcm transgene leads to an even further increase in the number of ectopic glia and in the proportion of glial cells that show Gcm autoregulation (the large majority if not all Repo(+) cells are βgal(+) as well: Fig. 1a,b,d ). Thus, gcm autoregulation is dosage dependent as is the potential to convert neurons in glia (see the number of neurons, Supplementary Fig. 1b–d ). 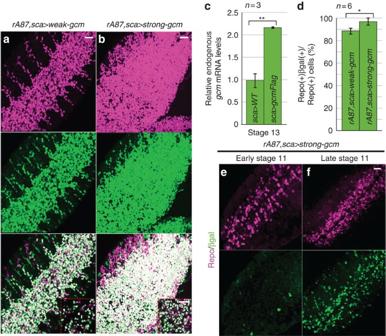Figure 1:gcm-positive autoregulation is Gcm dosage dependent. (a,b) Stage 16 embryos IHC for the nuclear glial marker Repo (magenta, unless specified) andgcmautoregulation marker (βgal, green, unless specified). All figures show confocal projections of ventral views, unless specified. Insets show magnifications of a region of interest, single sections. TheUAS-gcmline shown inawas used throughout the work, unless specified. (c) Mean levels of the endogenousgcmtranscripts insca>WT andsca>gcmFlagembryos (three qPCR assays, primers inSupplementary Table 1). (d) Percentage of Repo(+), βgal(+) cells in three segments of the embryonic VNC.n, number of embryos. (e,f) Repo and βgal expression at mentioned embryonic stages. In all figures: st, embryonic stages; error bars indicate±s.e.m.;P-value are estimated using student test and *P-value (0.05–0.01); **P-value (0.01–0.001); ***P-value <0.001; NS, nonsignificantP-value (>0.05); exact values for allP-values are detailed inSupplementary Note 1, scale bars, 20 μm. Figure 1: gcm- positive autoregulation is Gcm dosage dependent. ( a , b ) Stage 16 embryos IHC for the nuclear glial marker Repo (magenta, unless specified) and gcm autoregulation marker (βgal, green, unless specified). All figures show confocal projections of ventral views, unless specified. Insets show magnifications of a region of interest, single sections. The UAS - gcm line shown in a was used throughout the work, unless specified. ( c ) Mean levels of the endogenous gcm transcripts in sca> WT and sca>gcmFlag embryos (three qPCR assays, primers in Supplementary Table 1 ). ( d ) Percentage of Repo(+), βgal(+) cells in three segments of the embryonic VNC. n , number of embryos. ( e , f ) Repo and βgal expression at mentioned embryonic stages. In all figures: st, embryonic stages; error bars indicate±s.e.m. ; P -value are estimated using student test and * P -value (0.05–0.01); ** P -value (0.01–0.001); *** P -value <0.001; NS, nonsignificant P -value (>0.05); exact values for all P -values are detailed in Supplementary Note 1 , scale bars, 20 μm. Full size image We next asked whether the Gcm target Repo feeds back and controls gcm autoregulation, as suggested by the finding that ectopic βgal appears later than ectopic Repo ( Fig. 1e,f ). The levels of gcm RNA are indeed reduced in repo compared to wild-type (WT) embryos ( Fig. 2a ), as are the levels of βgal in a gcm rA87 repo background ( Supplementary Fig. 1e ). Similarly, gcm autoregulation is also reduced in gcm rA87 repo embryos ectopically expressing Gcm ( Fig. 2c ) compared with control embryos ( Fig. 2b ). 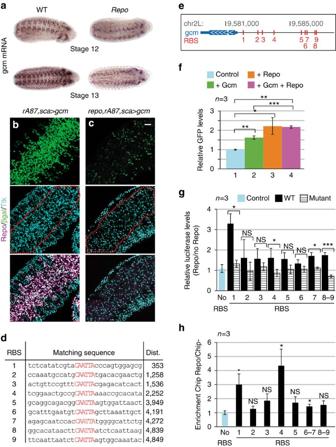Figure 2: Repo acts positively ongcmexpression. (a)In situhybridization with agcmprobe. (b)gcmrA87,sca>gcmand (c)repo,gcmrA87,sca>gcmst16 embryos IHC for Repo, βgal, Tramtrack (Ttk, cyan). Red dotted line: VNC. (d) Putative RBSs (in red) on the6kb-gcmpromoter. The first column indicates the RBS number, the second column the RBS sequence and the third column shows the distance of the RBS fromgcmtranscription start site. (e) Schematic of the genomic region containinggcmand its promoter. The RBSs are represented in red andgcmis indicated in blue. (f) Transcriptional effects of Gcm and Repo on thegcmpromoter. Mean GFP levels standardized against those of βgal (transfection control). WB on total protein extracts from cells transfected withp6kb-gcm-gal4+UAS-GFPwithout (column 1=control) or withpAct-gcmFlag,pAct-repoor both constructs, quantifications as inSupplementary Information. (g) Activation ofgcmpromoter’s RBSs by Repo. Mean luciferase levels standardized against those of βgal (transfection control). Luciferase activity was quantified from cells transfected with the indicatedpGL4.23_RBS, with or withoutpAct-repo.(h) Binding of Repo ongcmpromoter. qPCR on Repo ChIP to identify which RBSs in thegcmpromoter were pulled down with Repo in WT embryos at stage 11. Figure 2: Repo acts positively on gcm expression. ( a ) In situ hybridization with a gcm probe. ( b ) gcm rA87 ,sca>gcm and ( c ) repo,gcm rA87 ,sca>gcm st16 embryos IHC for Repo, βgal, Tramtrack (Ttk, cyan). Red dotted line: VNC. ( d ) Putative RBSs (in red) on the 6kb-gcm promoter. The first column indicates the RBS number, the second column the RBS sequence and the third column shows the distance of the RBS from gcm transcription start site. ( e ) Schematic of the genomic region containing gcm and its promoter. The RBSs are represented in red and gcm is indicated in blue. ( f ) Transcriptional effects of Gcm and Repo on the gcm promoter. Mean GFP levels standardized against those of βgal (transfection control). WB on total protein extracts from cells transfected with p6kb-gcm-gal4 + UAS-GFP without (column 1=control) or with pAct-gcmFlag , pAct-repo or both constructs, quantifications as in Supplementary Information . ( g ) Activation of gcm promoter’s RBSs by Repo. Mean luciferase levels standardized against those of βgal (transfection control). Luciferase activity was quantified from cells transfected with the indicated pGL4.23_RBS , with or without pAct-repo. ( h ) Binding of Repo on gcm promoter. qPCR on Repo ChIP to identify which RBSs in the gcm promoter were pulled down with Repo in WT embryos at stage 11. Full size image The positive effects of Repo may have at least three explanations: (1) Gcm needs Repo as a cofactor to act on its own promoter, (2) Repo directly binds the gcm promoter to activate it or (3) both processes contribute to induction. On transfecting Drosophila S2 cells, which express no endogenous gcm or repo , we found that Repo induces the expression of a reporter gene driven by the gcm promoter ( Fig. 2f columns 1,3), which contains nine Repo binding sites (RBS) [9] , [11] that are conserved in the Drosophila species (UCSC browser, http://genome.ucsc.edu/) ( Fig. 2d,e ). Each RBS was cloned in a luciferase reporter vector and co-transfected in S2 cells in the presence or absence of Repo (Sites 8–9 were cloned in the same vector, due to their close proximity). Repo induces significant expression of the luciferase reporters carrying RBS 1, 4, 7 8, 9 in their promoters ( Fig. 2g ). RBS 1 presents the strongest induction, with a 3.2 fold increase of the luciferase activity, comparable to previous results obtained with a luciferase reporter containing two RBS [11] . To assess in vivo the binding of Repo to the promoter of gcm , a ChIP targeting Repo was carried out in stage 11 WT embryos. RBS 1 and RBS 4 are significantly enriched, 3 and 4.2 folds respectively ( Fig. 2h ), at levels comparable to those obtained using the same approach on other transcription factors [17] , [18] , [19] . The other active sites seem moderately or not significantly enriched, which may be due to weak binding. Finally, none of the sites that are silent in S2 cells are enriched in our ChIP assay. In vitro experiments specifically performed on RBS 1 also confirm DNA binding ( Supplementary Fig. 1f ). Thus, Repo can directly bind the gcm promoter and maintains gcm expression. Repo promotes Gcm degradation via the proteasome Gcm may use its direct target Repo to reach the threshold levels required for gliogenesis. If that were the case, ectopic Repo expression should reinforce the gliogenic effects of gcm. Surprisingly, however, the number of gcm autoregulating cells on Repo and Gcm ectopic coexpression drastically decreases compared with that found in control embryos ( Fig. 3a,b bottom panels), as is the number of ectopic Repo(+) cells ( Fig. 3a,b top panels). Similar phenotypes were also obtained with the tagged transgene ( gcmFlag ) ( Supplementary Fig. 2a ) that allows discriminating endogenous from exogenous gcm expression. These effects are not due to Gal4 titration induced by using two reporters ( gcm+repo ) rather than one ( gcm ), since coexpression of green fluorescent protein (GFP) and Repo using the same driver does not reduce GFP expression ( Supplementary Fig. 2c–e ). Thus, Repo exerts opposite effects on gcm , and we speculated that Repo negatively controls gcm at posttranscriptional level. 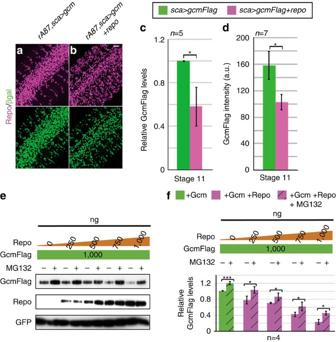Figure 3: Repo induces Gcm degradation. (a)gcmrA87,sca>gcmand (b) andgcmrA87,sca>gcm+repost16 embryos IHC for Repo and βgal. (c) Mean GcmFlag protein levels insca>GFP+gcmFlagandsca>GFP+gcmFlag+repoembryos, WB with α-Flag. In all WB on embryos, we used α-GFP as a loading control. Because the driver induces transient expression (Supplementary Fig. 2b), we used st11 embryos, which show peak levels ofgcm. (d) Quantification of GcmFlag intensity in embryos of the above genotypes (seeSupplementary Information). (e) GcmFlag protein degradation on Repo overexpression and treatment with MG132 proteasome inhibitor. WB on total protein extracts from transfected S2 cells using α-Flag for Gcm detection (upper part), α-Repo (middle part) and α-GFP (lower part). Unless specified, the transfection assays aiming at quantifying the Flag used GFP as loading and transfection control (pAct-gal4,pUAS-GFP). Quantification is shown in the histogram (f).n, number of assays. Figure 3: Repo induces Gcm degradation. ( a ) gcm rA87 ,sca>gcm and ( b ) and gcm rA87 ,sca>gcm+repo st16 embryos IHC for Repo and βgal. ( c ) Mean GcmFlag protein levels in sca>GFP+gcmFlag and sca>GFP+gcmFlag+repo embryos, WB with α-Flag. In all WB on embryos, we used α-GFP as a loading control. Because the driver induces transient expression ( Supplementary Fig. 2b ), we used st11 embryos, which show peak levels of gcm . ( d ) Quantification of GcmFlag intensity in embryos of the above genotypes (see Supplementary Information ). ( e ) GcmFlag protein degradation on Repo overexpression and treatment with MG132 proteasome inhibitor. WB on total protein extracts from transfected S2 cells using α-Flag for Gcm detection (upper part), α-Repo (middle part) and α-GFP (lower part). Unless specified, the transfection assays aiming at quantifying the Flag used GFP as loading and transfection control ( pAct-gal4 , pUAS-GFP ). Quantification is shown in the histogram ( f ). n , number of assays. Full size image Repo does not seem to affect gcm messenger RNA steady-state stability, as assessed by quantitative PCR (qPCR) analysis in sca>GFP+gcmFlag and in sca>GFP+gcmFlag+repo embryos. The levels of ectopic gcm transcripts, which do not depend on autoregulation, are similar in the two genotypes ( Supplementary Fig. 2g left columns). The levels of the endogenous transcripts are lower in sca>GFP+gcmFlag+repo than in sca>GFP+gcmFlag embryos ( Supplementary Fig. 2g right columns), suggesting that Repo negatively affects the Gcm/GcmFlag proteins and thereby autoregulation. To verify the role of Repo on the Gcm protein, we performed western blot (WB) analyses using embryos of the above genotypes at stage 11 ( Supplementary Fig. 2f , mid and left lanes), when Repo is already detected ( Supplementary Fig. S2d ). Gcm accumulates at lower levels in embryos ectopically coexpressing Gcm and Repo than in embryos that ectopically express only Gcm (histogram in Fig. 3c ), also confirmed by measuring total signal intensity on Flag immunohistochemistry (IHC) assays ( Fig. 3d ) [20] . No stable antibody against Gcm is currently available to monitor endogenous Gcm but the fact that the tag does not affect Gcm behaviour ( Supplementary Fig. 2a ) strongly suggests that the endogenous Gcm as well is destabilized and rapidly eliminated on Repo forced expression. Since the ubiquitin proteasome is involved in degrading many proteins including Gcm [21] , [22] , we asked whether Repo acts at least in part via this pathway. Gcm and Repo regulate their own expression and cross regulate, which makes it difficult to disentangle transcriptional from posttranscriptional regulation in embryos. We therefore transfected S2 cells with pAct-gcmFlag and pAct-repo expression constructs and found that Repo reduces Gcm levels in a dosage-dependent manner ( Fig. 3e,f ). We can exclude translation competition because Gcm and GFP cotransfection does not trigger the same effect. The above data also explain why the expression of the gcm reporter does not significantly increase in S2 cells coexpressing Repo and Gcm compared with those induced by the expression of Repo or Gcm alone ( Fig. 2f column 4 versus 2,3). Finally, treatment with the MG132 proteasome inhibitor alleviates the Repo-dependent decrease of Gcm levels ( Fig. 3e,f ). The partial rescue could be due to the fact that Repo-dependent but proteasome-independent pathways are also involved or that the levels of the inhibitor are not sufficient. Nevertheless, these results confirm that Repo affects Gcm levels via the proteasome. dCBP stabilizes Gcm The above data strongly suggest that Repo controls the timely decay of Gcm prompting us to ask what controls Gcm stabilization. Since in humans CBP/p300 acetylates and stabilizes hGCM1 (ref. 23 ), we assessed the effects of dCBP in cotransfection assays. dCBP clearly stabilizes GcmFlag ( Fig. 4a lanes 1–3, Supplementary Fig. 3a ) and the levels of GcmFlag significantly decrease on treatment with the CBP/p300 inhibitor C646 (ref. 24 ) ( Fig. 4a lanes 2–4, Supplementary Fig. 3a ). We further analysed the role of acetylation in Gcm stabilization by using the trichostatin (TSA) histone deacetylase (HDAC) inhibitor on cells transfected with a pAct-gcmFlag vector alone or with a pAct-repo construct ( Fig. 4b ). TSA treatment increases the levels of GcmFlag compared with those found in non-treated cells ( Fig. 4b lanes 1,2), indicating that the Gcm levels observed in a given cell are the net results of acetylating and deacetylating enzymes. Remarkably, TSA treatment allows the detection of Gcm even in the presence of Repo expression ( Fig. 4b lanes 3,4), suggesting that acetylation counteracts Repo-mediated Gcm degradation. The partial rescue could be due to the fact that the Repo-mediated degradation also involves HDACs that are not affected by TSA, which specifically targets class I and II families of enzymes but not class III HDACs [25] . Finally, the stabilizing effect of dCBP increases the transcriptional potential of Gcm, as dCBP–Gcm coexpression leads to a significant increase of reporter gene expression compared with that triggered by Gcm alone ( Fig. 4c ). 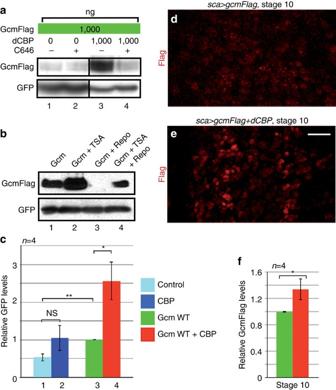Figure 4: dCBP stabilizes Gcm in the absence of Repo. (a) Effects of dCBP overexpression on GcmFlag stabilization and treatment with p300/CBP inhibitor C646. WB on total protein extracts from transfected S2 cells using α-Flag (upper lanes) and α-GFP (lower lanes). (b) Effects of HDACs on Gcm stability. WB on total protein extracts from cells transfected with the mentioned expression vectors and treated or not with TSA. (c) Transcriptional effects of Gcm and dCBP on the6kb-gcmpromoter. WB on total protein extracts on transfection withpAct-gcmFlag,pAct-dCBPor both constructs. Column 1 and GFP standardization as inFig. 2f. (d,e) α-Flag IHC on early embryos of the mentioned genotypes. (f) Mean Flag levels on WB from protein extracts ofsca>GFP+gcmFlagandsca>GFP+gcmFlag+dCBPembryos, normalized as above. Figure 4: dCBP stabilizes Gcm in the absence of Repo. ( a ) Effects of dCBP overexpression on GcmFlag stabilization and treatment with p300/CBP inhibitor C646. WB on total protein extracts from transfected S2 cells using α-Flag (upper lanes) and α-GFP (lower lanes). ( b ) Effects of HDACs on Gcm stability. WB on total protein extracts from cells transfected with the mentioned expression vectors and treated or not with TSA. ( c ) Transcriptional effects of Gcm and dCBP on the 6kb-gcm promoter. WB on total protein extracts on transfection with pAct-gcmFlag , pAct-dCBP or both constructs. Column 1 and GFP standardization as in Fig. 2f . ( d , e ) α-Flag IHC on early embryos of the mentioned genotypes. ( f ) Mean Flag levels on WB from protein extracts of sca>GFP+gcmFlag and sca>GFP+gcmFlag+dCBP embryos, normalized as above. Full size image In a more functional perspective, we compared embryos ectopically coexpressing GcmFlag and dCBP to those that ectopically express only GcmFlag. To exclude any negative effect played by Repo, we analysed stage 10 embryos, which do not express Repo yet ( Supplementary Fig. 3b,c ). WB and IHC analyses show a significant increase of GcmFlag protein levels in embryos coexpressing GcmFlag and dCBP compared with those found in embryos that only ectopically express GcmFlag ( Fig. 4d–f ). In sum, dCBP stabilizes Gcm and increases its transcriptional activity. dCBP acetylates Gcm Since dCBP acetylates several proteins and histone tails, we asked whether the effects of dCBP on Gcm are direct. We first scored for protein–protein interaction. Drosophila and mammalian Gcm proteins show conservation in the domain of hGCM1-CBP physical interaction ( Fig. 5a pink boxed sequences) that triggers hGCM1 acetylation [26] . Immunoprecipitation (IP) assays on transfecting the GcmFlag expression vector show that Gcm and dCBP also interact ( Fig. 5c top panel). We next scored for dCBP-mediated acetylation. Gcm contains 18 predicted acetylated lysines (K) via CBP/p300 HAT family (ASEB, acetylation set enrichment-based), several of which are conserved throughout evolution and have a high probability of acetylation ( P <0.05) ( Fig. 5b ). We transfected the pAct-gcmFlag vector alone or with dCBP and performed an IP with α-acetyl K (α-Ac): a signal corresponding to the expected GcmFlag molecular weight was specifically detected on the extracts from the Gcm–dCBP expressing cells ( Fig. 5c Middle panel). In the same transfection conditions, we performed the IP with α-Flag and WB with α-Ac ( Fig. 5c bottom panel lower lanes) and showed that a fraction of GcmFlag is acetylated ( Fig. 5c bottom panel upper lanes). The lack of acetylated Gcm on co-IP from S2 cells only expressing Gcm, even though dCBP is endogenously expressed, may be due to the percentage of acetylated Gcm, to dynamic acetylation states and/or to the amount of Gcm present in the total extract used for the IP, too low to be detected by this analysis (see below). 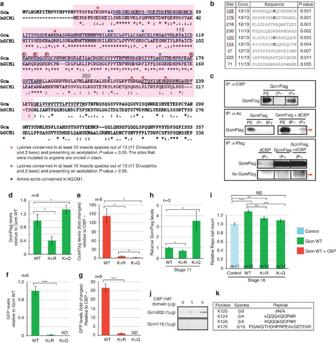Figure 5: Mutation of Gcm acetylation sites prevent its stabilization by CBP. (a) Amino-acid sequence alignment of hGCM1 and Gcm. Pink box: region essential for CBP and hGCM1 binding; DBD in blue; the PEST domain in black; NLS in magenta. (b) Gcm lysines predicted to be acetylated. Second column: Conservation in 13 insect species; fourth column:P-value of acetylation prediction, only sites withP-value <0.05 are notified. Mutagenized lysines are in bold. (c) Gcm–dCBP interaction: IP with α-dCBP, α-Ac, α-Flag on protein lysates. Top panel: Transfection withpAct-gcmFlagIP with (IP+) or without (IP−) α-dCBP, PE (protein extract)=input, WB with α-Flag. Middle panel: Transfection withpAct-gcmFlag, with (right lanes) or without (left lanes)pAct-dCBP, IP with/without α-acetyl K (α-Ac), WB with α-Flag. Red arrow: acetylated GcmFlag. Bottom panel: Transfection as above, IP with/without α-Flag, WB with α-Flag, to reveal the total amounts of Gcm (upper lanes) and with α-Ac (lower lanes). Red arrow, as above. (d) Mean Flag levels in cells transfected with WT or mutant (K>R, K>Q)gcmFlag. Values are relative to those of the WT. (e) Same WB analysis as in (d), in the presence ofpAct-dCBP. Values indicate fold-changes compared with transfection withoutpAct-dCBP(CBP−). (f) Transcriptional effects of WT and mutant Gcm as in (d), mean GFP levels relative to those of the WT. ND, undetectable levels. (g) Same WB analysis as inf, in the presence ofpAct-dCBP. Values indicate fold-changes compared with those obtained withoutpAct-dCBP. (h) WB showing the mean Flag levels in embryos ectopically expressing WT or mutant GcmFlag, normalized as above. (i) Number of Repo(+) cells in five segments from the VNC ofnembryos. Values expressed as relative to the number of Repo(+) cells of WT embryos (light blue, control column). (j) WB targeting acetylated lysines in Gcm202 or Gcm115 acetylatedin vitrowith a gradient of dCBP HAT. (k) Mass spectrometry analysis of K120, K124, K128 and K179 of the acetylated Gcm202. Second column: Number of spectra presenting acetylation/total number of spectra covering the K (only high confidence spectra were used), third column: sequenced peptides. Figure 5: Mutation of Gcm acetylation sites prevent its stabilization by CBP. ( a ) Amino-acid sequence alignment of hGCM1 and Gcm. Pink box: region essential for CBP and hGCM1 binding; DBD in blue; the PEST domain in black; NLS in magenta. ( b ) Gcm lysines predicted to be acetylated. Second column: Conservation in 13 insect species; fourth column: P -value of acetylation prediction, only sites with P -value <0.05 are notified. Mutagenized lysines are in bold. ( c ) Gcm–dCBP interaction: IP with α-dCBP, α-Ac, α-Flag on protein lysates. Top panel: Transfection with pAct-gcmFlag IP with (IP+) or without (IP−) α-dCBP, PE (protein extract)=input, WB with α-Flag. Middle panel: Transfection with pAct-gcmFlag , with (right lanes) or without (left lanes) pAct-dCBP , IP with/without α-acetyl K (α-Ac), WB with α-Flag. Red arrow: acetylated GcmFlag. Bottom panel: Transfection as above, IP with/without α-Flag, WB with α-Flag, to reveal the total amounts of Gcm (upper lanes) and with α-Ac (lower lanes). Red arrow, as above. ( d ) Mean Flag levels in cells transfected with WT or mutant (K>R, K>Q) gcmFlag . Values are relative to those of the WT. ( e ) Same WB analysis as in ( d ), in the presence of pAct-dCBP . Values indicate fold-changes compared with transfection without pAct-dCBP (CBP−). ( f ) Transcriptional effects of WT and mutant Gcm as in ( d ), mean GFP levels relative to those of the WT. ND, undetectable levels. ( g ) Same WB analysis as in f , in the presence of pAct-dCBP . Values indicate fold-changes compared with those obtained without pAct-dCBP . ( h ) WB showing the mean Flag levels in embryos ectopically expressing WT or mutant GcmFlag, normalized as above. ( i ) Number of Repo(+) cells in five segments from the VNC of n embryos. Values expressed as relative to the number of Repo(+) cells of WT embryos (light blue, control column). ( j ) WB targeting acetylated lysines in Gcm202 or Gcm115 acetylated in vitro with a gradient of dCBP HAT. ( k ) Mass spectrometry analysis of K120, K124, K128 and K179 of the acetylated Gcm202. Second column: Number of spectra presenting acetylation/total number of spectra covering the K (only high confidence spectra were used), third column: sequenced peptides. Full size image Following this, we assessed the relevance of Gcm acetylation by mutagenesis. To preserve as much as possible the overall protein structure, we limited the mutagenesis to four K residues that present: (i) highest acetylation potential, (ii) most conserved amongst the thirteen insect species for which the genome is available, (iii) presence in hGCM1 ( Fig. 5a red encircled asterisks, Fig. 5b sites in bold). We substituted them with arginine (R) residues, as a mimic of not-acetylated K, and found that the stability of the transfected mutant protein (GcmFlag K>R) severely decreases ( Fig. 5d ). Furthermore, the transactivation potential of this protein is much weaker than that of the WT one ( Fig. 5f ). Finally, we tested the impact of acetylation in vivo , using transgenic flies that carry a WT or a K>R UAS–gcmFlag construct inserted at the same genomic site, thus avoiding position effects and differences in the expression levels. We crossed the flies with the sca-gal4 driver and validated the cell culture data: the WT protein accumulates more ( Fig. 5h ) and induces more glia ( Fig. 5i ) than the mutant one, formally demonstrating that acetylation is important for Gcm stability and for gliogenesis. Interestingly, the mutant protein is still stabilized and its transcriptional activity is still potentiated by dCBP, albeit at much lower levels than the WT one ( Fig. 5e,g ). The mutant protein is also partially active in vivo . Thus, other acetylated residues may be relevant as well and/or that other modifications control Gcm activity. In addition, we mutagenized the same four K sites to glutamine (Q), which in some cases is considered as an acetylation mimicking mutation [27] , [28] , expecting a stabilization of the Gcm protein. The mutant protein (GcmFlag K>Q) does accumulate at higher levels compared with the WT, in transfection assays ( Fig. 5d ). Strikingly, however, it is completely transcriptionally inactive ( Fig. 5f ), likely due to alteration of the DNA binding property of Gcm, as Q displays different charge and length compared with K [28] . The presence of dCBP barely changes the levels of the K>Q protein and does not render it transcriptionally active ( Fig. 5e,g ). Finally, ectopic expression of a K>Q-targeted transgene shows that the mutations also stabilize the protein and render it inactive in vivo ( Fig. 5h,i ). To formally demonstrate dCBP-dependent acetylation and identify the acetylated K residue(s), we carried out in vitro assays. Two constructs were used, one expressing the first 115 amino acids of the Gcm–DBD (Gcm115) and one extending to amino acid 202 (Gcm202) ( Fig. 5a ). Only the latter contains the four lysines highly conserved in insect and mammals and predicted to be acetylated: K120, K124, K128 and K179. The WB targeting acetyl lysines revealed that only Gcm202 can be acetylated by dCBP, strongly suggesting that at least one of the four conserved K is acetylated by dCBP, in a dosage-dependent manner ( Fig. 5j ). Finally, mass spectrometry analysis of the acetylated Gcm202 product clearly demonstrated the acetylation of K128. For the other residues, the current MS techniques are not sufficiently sensitive: K120 was not covered by the analysis; therefore, the acetylation state could not be assessed; K124 was poorly covered and the lateral position of the residue is suboptimal for detecting acetylation; K179, the most covered lysine in the analysis, may still be weakly acetylated ( Fig. 5k ). The in vitro data nevertheless allow us to demonstrate formally that Gcm is acetylated by dCBP, at the resolution of a single lysine residue, K128. In sum, we show that dCBP acetylates Gcm, that the state of Gcm acetylation regulates its levels and activity, and, importantly, that this controls gliogenesis. dCBP enhances Gcm degradation in the presence of Repo The opposite effects of dCBP and Repo on Gcm led us to analyse the tripartite interaction and its possible role on the dynamics of Gcm accumulation. We transfected cells with pAct-gcmFlag and pAct-repo vectors with or without pAct-dCBP . Since the negative effect of Repo on GcmFlag is strong and dosage dependent, we used a ratio of one dose of pAct-repo against two doses of pAct-gcmFlag and we analysed three conditions: low, medium and high Gcm/Repo expression levels ( Fig. 6a columns 1–4, 5–8, 9–12, respectively). Keeping constant the ratio between Gcm and Repo (2:1) allowed us to focus on the impact of absolute protein levels. 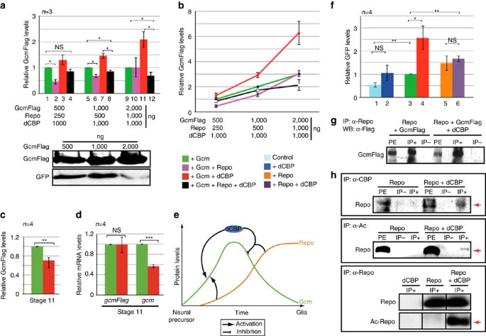Figure 6: dCBP enhances Repo-mediated Gcm degradation. (a) Top panel: Flag levels in transfected cells as mentioned in the color-coding legend. All values are relative to those of cells only transfected withpAct-gcmFlag(green columns). Mean of three WB normalized as above. Bottom panel: WB showing the Flag levels on transfecting increasing amounts ofpAct-gcmFlag. (b) Graphical representation of the data ina. Note that here the Flag levels are only normalized against those of GFP. (c) Mean Flag levels on WB from protein extracts ofsca>GFP+gcmFlagandsca>GFP+gcmFlag+dCBPembryos, normalized as above. (d) Mean levels of endogenous (right two columns) and ectopicgcmtranscripts (gcmFlag, left two columns) insca>GFP+gcmFlagandsca>GFP+gcmFlag+dCBP, four qPCR assays. (e) Schematics summarizing the regulatory network. (f) Transcriptional effects of dCBP, Gcm and Repo on the6kb-gcmpromoter. WB on total protein extracts on transfection withpAct-gcmFlag,pAct-repo, pAct-dCBPalone or in combination. The rest as inFig. 2f. The first two lanes are the same as those inFig. 4c. (g) Repo–Gcm interaction with/without dCBP. Protein lysates prepared from cells transfected with the mentioned vectors were subjected to IP with/without α-Repo, WB with α-Flag. (h) Repo-dCBP interaction: IP with α-dCBP, α-Ac, α-Repo on protein lysates from cells transfected withpAct-repowith/withoutpAct-dCBP.Symbols as inFig. 5c. Top panel: IP with/without α-dCBP, WB with α-Repo (red arrow indicates the Repo product). Middle panel: IP with/without α-Ac, WB with α-Repo. Red arrow indicates acetylated Repo. Bottom panel: IP with/without α-Repo, WB with α-Repo (upper lanes) and α-Ac (lower lanes). Figure 6: dCBP enhances Repo-mediated Gcm degradation. ( a ) Top panel: Flag levels in transfected cells as mentioned in the color-coding legend. All values are relative to those of cells only transfected with pAct-gcmFlag (green columns). Mean of three WB normalized as above. Bottom panel: WB showing the Flag levels on transfecting increasing amounts of pAct-gcmFlag . ( b ) Graphical representation of the data in a . Note that here the Flag levels are only normalized against those of GFP. ( c ) Mean Flag levels on WB from protein extracts of sca>GFP+gcmFlag and sca>GFP+gcmFlag+dCBP embryos, normalized as above. ( d ) Mean levels of endogenous (right two columns) and ectopic gcm transcripts ( gcmFlag , left two columns) in sca>GFP+gcmFlag and sca>GFP+gcmFlag+dCBP , four qPCR assays. ( e ) Schematics summarizing the regulatory network. ( f ) Transcriptional effects of dCBP, Gcm and Repo on the 6kb-gcm promoter. WB on total protein extracts on transfection with pAct-gcmFlag , pAct-repo, pAct-dCBP alone or in combination. The rest as in Fig. 2f . The first two lanes are the same as those in Fig. 4c . ( g ) Repo–Gcm interaction with/without dCBP. Protein lysates prepared from cells transfected with the mentioned vectors were subjected to IP with/without α-Repo, WB with α-Flag. ( h ) Repo-dCBP interaction: IP with α-dCBP, α-Ac, α-Repo on protein lysates from cells transfected with pAct-repo with/without pAct-dCBP. Symbols as in Fig. 5c . Top panel: IP with/without α-dCBP, WB with α-Repo (red arrow indicates the Repo product). Middle panel: IP with/without α-Ac, WB with α-Repo. Red arrow indicates acetylated Repo. Bottom panel: IP with/without α-Repo, WB with α-Repo (upper lanes) and α-Ac (lower lanes). Full size image At Low levels of Gcm and Repo, Gcm is degraded, however, as the amounts of the two proteins increases, Gcm is less degraded (compare green and pink columns at the three concentration conditions in Fig. 6a ). This suggests that Gcm and Repo compete for a limiting factor. At low levels of Repo and Gcm, the factor is abundant and Repo efficiently degrades Gcm ( Fig. 6a columns 1,2) whereas, at high levels, the factor becomes limiting and Repo no longer degrades Gcm efficiently ( Fig. 6a columns 9,10). The cotransfection assays suggest that dCBP corresponds to the limiting factor ( Fig. 6a compare pink and black columns). In the low-level condition, dCBP overexpression partially rescues the negative effect of Repo ( Fig. 6a columns 1–4). Thus, dCBP prevents Repo-mediated Gcm degradation. In the medium-level condition, adding dCBP does not seem to rescue the effects of Repo and Gcm levels are decreased compared with Gcm alone transfection ( Fig. 6a columns 5–8). Interestingly, in the high-level condition, the effects of dCBP are reversed so that it enhances Gcm degradation in the presence of Repo ( Fig. 6a columns 9–12, Fig. 6b compare the behaviour of black, pink lines and red line). Thus, Gcm levels are controlled by a tight equilibrium between Gcm and Repo proteins ( Fig. 6b ). In sum, the dCBP limiting factor acts positively on the two proteins, thereby triggering opposite effects: direct Gcm stabilization and indirect Gcm destabilization mediated by Repo. We next analysed stage 11 embryos and tested whether dCBP enhances Gcm degradation in the presence of Repo in vivo : animals ectopically coexpressing GcmFlag–dCBP show a significant decrease in the GcmFlag levels compared with those that ectopically express only GcmFlag ( Fig. 6c and Supplementary Fig. 2f right lane). The decrease of GcmFlag accumulation is not caused by defects in gcmFlag transcripts, whose amounts are similar in the two genotypes ( Fig. 6d left two columns). As expected, the endogenous gcm transcripts show significant reduction in the presence of ectopically expressed dCBP ( Fig. 6d right two columns), likely due to the negative control of gcm autoregulation. Finally, the negative effects of dCBP could also be explained at least in part by the fact that Gcm and Repo may both need dCBP and compete for their transcriptional activity. Cotransfection assays, however, show that dCBP affects the transcriptional activity of Gcm (enhancement) but not that of Repo, nor does it affect Repo stability ( Fig. 6f compare columns 3–4 and 5–6, Supplementary Fig. 3d ). The in vivo and the S2 cell data fit well with the dynamic accumulation and the levels of Gcm and Repo observed during gliogenesis (see model in Fig. 6e ). At the beginning, Gcm starts accumulating and rapidly reaches threshold levels, via the positive transcriptional and posttranscriptional contribution of dCBP. Gcm then activates target genes including Repo and itself, so that both Repo and Gcm help building up each other’s transcription. As high Gcm and Repo levels are reached, dCBP facilitates Repo-mediated Gcm destruction and Gcm fades away, while Repo stays on. This allows terminal glial differentiation. dCBP facilitates Repo–Gcm interaction The above data suggest that Repo counteracts Gcm stability by sequestering dCBP and that it destabilizes Gcm more efficiently in the presence of dCBP. If so, Repo should interact physically with dCBP and Gcm. IP assays in cells overexpressing Repo alone or together with dCBP reveals that the two proteins interact in cells ( Fig. 6h top panel) and the complex was also detected in embryos overexpressing Gcm ( Supplementary Fig. 3e : IP α-Repo, WB α-CBP and vice versa). Repo also directly associates with Gcm ( Fig. 6g , left side, IP assays using the α-Flag on S2 cells expressing Repo and GcmFlag, note that we used the proteasome inhibitor MG132 to counteract the destabilizing effects of Repo on Gcm). In these conditions, simultaneous dCBP coexpression does not disrupt Repo–Gcm interaction ( Fig. 6g , right side). Rather, dCBP may facilitate Repo–Gcm interaction and increase the ability of Repo to degrade Gcm (compare the relative intensity of the signals on IP and in the input to those obtained in the absence of dCBP, cells treated in parallel). This is also in line with the WB data ( Fig. 6a,b ). Together with the fact that acetylation may enhance protein–protein interaction [29] , these data led us to assess whether dCBP mediates the acetylation of Repo, which contains twenty-seven putative sites, more than fifteen showing a high probability of acetylation and being conserved throughout the thirteen insect genomes ( Supplementary Fig. 3f red asterisks). An IP assay for acetylated proteins in cells expressing Repo with or without dCBP shows that dCBP does mediate Repo acetylation ( Fig. 6h middle and bottom panels). In sum, dCBP and Repo are shared components of two interlocked loops ( Fig. 6e ): on the one hand dCBP induces Gcm stability, while helping Repo-induced Gcm degradation; on the other hand, Repo induces gcm expression while mediating Gcm degradation. dCBP-forced expression inhibits gliogenesis and promotes neuronal differentiation We next analysed the in vivo relevance of the outlined network. First, we assessed the impact of dCBP levels on endogenous glia. sca>dCBP embryos contain the same number of glia as sca> WT ( Fig. 7a ) and dCBP mutant ( nej ) embryos [30] . Thus, gliogenesis tolerates fluctuations in the amounts of dCBP. Because of the maternal dCBP component ( Supplementary Fig. 4a–f ) and because the whole cascade relies on positive and negative interconnected loops, we used sensitized backgrounds to alter the relative and the absolute amounts of dCBP and/or Gcm. In these conditions, increasing and decreasing dCBP levels aggravates and rescues the gcm loss of function phenotype, respectively; thus, dCBP represses gliogenesis. Typically, gcm heterozygous embryos are like WT embryos, but if they overexpress dCBP, they show fewer glia ( Fig. 7a columns 1–4). Furthermore, dCBP overexpression further reduces the number of glia observed in gcm hypomorphic homozygous embryos ( Fig. 7a columns 5,6). Similarly, lack of dCBP alleviates the phenotype due to gcm hypomorphic mutations ( Fig. 7a columns 7,8). The same applies to ectopic glia. The number of ectopic Repo(+) cells is significantly reduced in sca>gcm+dCBP compared with that found in sca>gcm control embryos ( Fig. 7 columns 9,10). In agreement with the hypothesis that altering the Gcm:dCBP ratio breaks the homeostasis, the above phenotypes are dosage dependent ( Supplementary Fig. 4k–m ). Since dCBP also affects later steps of glial differentiation [31] , [32] , we confirmed the early phenotype by analysing a specific lineage. Introducing a gcm transgene carrying its 2 kb promoter region in a gcm -null background is sufficient to rescue the birth of the so-called NB1-1 glia [12] ; however, gcm -mutant embryos carrying the transgene and expressing high dCBP levels show no rescue ( Supplementary Fig. 4g–i ). 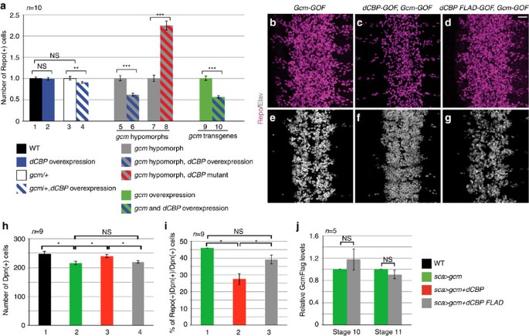Figure 7: dCBP HAT inhibits gliogenesis and promotes neuronal differentiation. (a) Number of Repo(+) cells in three segments from the VNC of st16 embryos mutant or ectopically expressinggcmand/or dCBP.n, number of embryos. Note that the absolute number of glia ingcm-mutant or overexpressing embryos (grey columns and green column) differs from that of WT embryos (black column). In the genotypes considered as controls, however, the number of glia is brought to 1, for the sake of simplicity. Genotypes as inSupplementary Information. (b–g) St16 embryos IHC for Repo and Elav. (h) Number of Dpn(+) cells in the VNC of st12 embryos and that of Repo(+), Dpn(+) cells ini. (j) Mean Flag levels on WB from embryonic extracts of the mentioned genotypes and stages, normalized as above.n, number of assays. Figure 7: dCBP HAT inhibits gliogenesis and promotes neuronal differentiation. ( a ) Number of Repo(+) cells in three segments from the VNC of st16 embryos mutant or ectopically expressing gcm and/or dCBP. n , number of embryos. Note that the absolute number of glia in gcm -mutant or overexpressing embryos (grey columns and green column) differs from that of WT embryos (black column). In the genotypes considered as controls, however, the number of glia is brought to 1, for the sake of simplicity. Genotypes as in Supplementary Information . ( b – g ) St16 embryos IHC for Repo and Elav. ( h ) Number of Dpn(+) cells in the VNC of st12 embryos and that of Repo(+), Dpn(+) cells in i . ( j ) Mean Flag levels on WB from embryonic extracts of the mentioned genotypes and stages, normalized as above. n , number of assays. Full size image We then assessed how does dCBP affect gliogenesis and found that it impacts on Gcm autoregulation, an important step in the Gcm pathway [4] , [12] , [33] , as the percentage of cells showing gcm autoregulation decreases significantly when Gcm and dCBP are ectopically coexpressed ( Supplementary Fig. 4j ). Since ectopic Gcm works by converting neural stem cells into glia [31] , we analysed the effects of dCBP on this process using the NB marker Deadpan (Dpn). The number of Dpn(+) cells decreases on Gcm expression ( Fig. 7h compare black and green columns) and this phenotype is rescued on Gcm–dCBP coexpression ( Fig. 7h red column). Similarly, the number of Dpn(+), Repo(+) NBs, that is, on their way to adopt the glial fate, also decreases on Gcm–dCBP coexpression ( Fig. 7i compare red and green columns). Thus, dCBP prevents the ability of Gcm to convert NBs into glia. In line with this (and with the fact that there is less Gcm when dCBP is coexpressed, Fig. 6c ) dCBP favors the neuronal programme: sca>gcm+dCBP embryos show a higher number of neurons than sca>gcmFlag embryos ( Fig. 7b,c,e,f ). Thus, dCBP promotes neurogenesis and represses gliogenesis in the multipotent precursors. Finally, the acetyltransferase activity of dCBP is required, as none of the above phenotypes (number of glia, neurons, NBs and that of NB on their way to become glia) was observed in coexpression experiments with Gcm and a mutant dCBP transgene (dead HAT dCBP or FLAD [30] ) ( Fig. 7d,g–i ). Importantly, dCBP FLAD expression does not affect Gcm stability in vivo ( Fig. 7j ). In sum, the dCBP HAT allows Gcm to produce the appropriate number of glia and neurons from multipotent precursors. Cell fate building involves an intermediate transient state The above data show that timely regulation of Gcm controls lineage progression, the event that leads to glial specification. To complete our analysis, we asked whether dCBP affects the very first step of glial specification, that is, the initial choice between the glial and the neuronal fates. Interestingly, forced expression of dCBP induces a rare but fully penetrant phenotype that is absent in WT mature embryos: the coexpression of glial and neuronal markers ( Fig. 8a ). This suggests that Gcm is expressed below threshold levels, which induces Repo expression very poorly, hence producing cells in which the glial fate cannot be stably implemented and the neuronal fate cannot be stably repressed. Of note, this phenotype also occurs in (few) supernumerary glia induced that likely express ectopic Gcm at suboptimal levels ( Fig. 8b ). The presence of cells in an intermediate neuronal–glial fate suggests there may also be cells that take the glial fate transiently but then revert to neurons. To prove this, we generated a lineage tracer that would allow us to follow all glial cells. 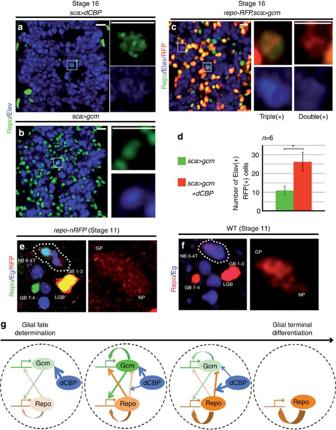Figure 8: Glial specification and intermediate fates. (a,b) Optical sections ofsca>dCBP(a) andsca>gcm(b) embryos showing cells weakly coexpressing Repo (green) and Elav. (c) Optical section of Gcm overexpressing embryo carrying therepo-RFPglial lineage tracer and labelled for Repo, Elav and RFP. Note the presence of Repo(+), Elav(+), RFP(+) (triple(+)) and Elav(+), RFP(+) cells (double(+)). (d) Number of Elav(+), RFP(+) cells in the whole VNC of st16 embryos. (e)repo-RFPembryos labelled with the NB lineage-specific marker Eagle (Eg), Repo and the glial lineage tracer RFP. Dotted line: progenies of the NB6-4T lineage. LGB, GB7-4 and GB1-3 indicate other glial lineages, NP and GP, respectively. (f) WT embryos labelled with Eg and Repo. Dotted line: As above. (g) Detailed sequence of the tripartite interaction. Line and horizontal arrow: Gene and transcription start site, respectively; ellipse: protein; arrow: positive effect; blocked arrow: negative effect. Figure 8: Glial specification and intermediate fates. ( a , b ) Optical sections of sca>dCBP ( a ) and sca>gcm ( b ) embryos showing cells weakly coexpressing Repo (green) and Elav. ( c ) Optical section of Gcm overexpressing embryo carrying the repo-RFP glial lineage tracer and labelled for Repo, Elav and RFP. Note the presence of Repo(+), Elav(+), RFP(+) (triple(+)) and Elav(+), RFP(+) cells (double(+)). ( d ) Number of Elav(+), RFP(+) cells in the whole VNC of st16 embryos. ( e ) repo-RFP embryos labelled with the NB lineage-specific marker Eagle (Eg), Repo and the glial lineage tracer RFP. Dotted line: progenies of the NB6-4T lineage. LGB, GB7-4 and GB1-3 indicate other glial lineages, NP and GP, respectively. ( f ) WT embryos labelled with Eg and Repo. Dotted line: As above. ( g ) Detailed sequence of the tripartite interaction. Line and horizontal arrow: Gene and transcription start site, respectively; ellipse: protein; arrow: positive effect; blocked arrow: negative effect. Full size image repo-RFP flies express the stable RFP protein under the control of a repo promoter that faithfully reproduces the repo expression profile [34] . RFP is detectable earlier than Repo and later on the two labelling colocalize ( Supplementary Fig. 5b ). On ectopic Gcm expression, numerous cells display the intermediate fate (triple(+): (Elav(+),RFP(+),Repo(+), white arrowheads) or revert to neurons ((double(+): Elav(+),RFP(+), empty arrowheads) ( Supplementary Fig. 5a ). These phenotypes are also detected at late stages, albeit less numerous ( Fig. 8c ; Supplementary Fig. 5c ). Thus, repo-RFP identifies cells that have adopted a stable or a transient glial fate. Interestingly, Gcm–dCBP coexpression enhances the number of presumptive glia that have reverted to neurons cells compared with that found in sca>gcm embryos ( Fig. 8c,d ). Accordingly, the total number of RFP(+) cells and that of Repo(+) alone decreases ( Supplementary Fig. 5d ). Finally, we asked whether the ‘frozen’ intermediate fate reflects a situation that occurs transiently during development. The multipotent precursor NB6-4T divides and produces a neuronal precursor (NP) that accumulates gcm transcripts at very low levels, and a glial precursor (GP) that accumulates it at high levels [35] , [36] . The NP expresses the repo-RFP reporter and, more importantly, the Repo protein itself, in a transient manner and at low levels ( Fig. 8e,f ). Thus, the NP initially expresses an intermediate fate that is normally rapidly suppressed, to give rise to a stable neuronal fate. In sum, dCBP contributes to the acquisition of the glial fate. Multipotency and lineage specification are the forces that control the generation of specific, stable, fates at the correct number, place and time. We here show that two interlocked and opposing loops control the establishment of the glial fate in the Drosophila nervous system. These homeostatic and dynamic processes are triggered by the fate determinant itself, hence ensuring efficient and robust glial differentiation. While different levels of transcription factors are known to trigger specific fates [24] , [37] , [38] , we here identify temporal regulation as an additional important step. The core of the network is a Gcm–Repo feedback loop. At early stages, the fate determinant Gcm is positively regulated. It induces the expression of the homeodomain protein Repo, which feeds back positively onto gcm expression as does Gcm itself. In addition, dCBP stabilizes Gcm via acetylation, similar to the activity of CBP/p300 on other transcription factors, including p53, c-Myc and hGCM1 (refs 23 , 39 ). The relevance of Gcm acetylation is also highlighted by the stabilizing effects of the HDAC inhibitor and formally demonstrated by mutagenesis of the acetylation sites. As the Repo protein accumulates, the ratio between the two molecules and their absolute levels change; Repo starts exerting a negative effect on the Gcm protein. Repo represents the ideal trigger of Gcm degradation since (i) it is a Gcm direct target, (ii) is continuously expressed in all glia, (iii) it positively autoregulates, hence becoming independent of Gcm and, finally, (iv) its lack prevents glial terminal differentiation. The role of transcription factors on stimulating the degradation of other factors just starts to emerge. To our knowledge, the only report describing a similar effect concerns the transcription factor STAT2, activated by inflammatory signals, which enhances the proteasomal degradation of RCAN1 (regulator of calcineurin) through the ubiquitin E3 ligase FBW7 (ref. 40 ). dCBP enhances the negative effect of Repo on Gcm in cells and in vivo . Since dCBP (i) forms a complex with Repo and Gcm, (ii) mediates Repo and Gcm acetylation, (iii) enhances Repo–Gcm interaction as does the inhibition of deacetylation, we speculate that Repo acetylation is necessary for its interaction with Gcm, which then triggers Gcm degradation. This goes along with the findings that dCBP increases Gcm accumulation at stages at which Repo is not expressed and decreases it at stages of Gcm–Repo coexpression. Thus, homeostatic interactions sequentially move the balance from positive to negative effects and from transcriptional to posttranscriptional pathways. As a consequence, gcm expression fades away while repo is stably expressed and executes the glial terminal differentiation programme. Disrupting the network affects the number of neurons and glia, in line with the dosage dependence of the gcm loss and gain of function phenotypes. The timely control of Gcm stability emerges as an efficient and fast strategy to produce a robust fate, since the determinant causes its own destruction once it has triggered the novel transcriptional programme. Several mechanisms may account for our findings. (i) Repo may prevent Gcm stability by competing for the same dCBP domain, similar to the competition between STAT2 and p65 for the control of tumour necrosis [41] . The idea that dCBP represent a limiting factor is in line with the haploinsufficient phenotype observed in humans [15] . (ii) Repo may interact with HDACs that modify and prompt Gcm for degradation. (iii) Repo may interact with E3 ubiquitin ligases. The F-box protein β-TrCP is a p300 interactor [42] and Ago as well as Slimb, the fly β-TrCP ortholog, mediate Gcm degradation via the proteasome [21] . Regardless of the specific pathway involved, the analysis of discrete phenotypes and sensitized backgrounds combined with the in vitro assays allowed us to identify transcriptional and posttranscriptional feedback loops that are otherwise difficult to dissect. Based on all data, we propose a model for the acquisition of the glial fate ( Fig. 8g ). In addition to affecting the number of neurons and glia, altering the interconnected loops generates stable intermediate neuronal/glial fates, a phenotype that was observed in metastatic brain tumours [43] , implying that ambiguous fates may represent a signature of cancer cells. Interestingly, the intermediate phenotype occurs transiently in natural conditions in the neuronal progeny issued from the neuroGPs. The little amount of Gcm present in these cells is likely eliminated by Repo, thereby producing the neuronal fate. Of note, the neuronal protein Elav was described as being transiently expressed in all embryonic glial lineages at early stages [44] , suggesting that an analogous process occurs in the glial progeny. Hence, bidirectional interactions and balance between a fate determinant, its target and a widely expressed HAT ensure the dynamic levels of Gcm that induces a stable glial identity. Interestingly, the so-called epithelial–mesenchymal transition (EMT), which triggers heart morphogenesis, mesoderm and neural crest formation in vertebrates, also involves intermediate, transient, phenotypes referred to as metastable states [45] . EMT depends on transcription factors including Twist and Snail, whose activity is quantitatively regulated at the level of protein stability [46] , [47] . Little is known about how the transiently expressed Twist protein regulates EMT during embryonic development. Interestingly, however, Drosophila Twist triggers the mesodermal fate, which is stabilized by the evolutionarily conserved dMef2 protein [48] . This homeodomain containing protein and Twist cross and autoregulate transcriptionally. Given that vertebrate Twist is highly expressed in tumours and has an essential role in metastasis [49] , it will be interesting to determine whether a homeostatic balance similar to the one working in the Gcm pathway also applies to Twist. In sum, our work identifies the molecular pathway controlling glial specification, paving the way for future work on other developmental pathways. Understanding whether intermediate states have been underscored due to their transient nature may clarify pathological phenotypes such as those observed in cancer. Drosophila strains w 1118 was the WT. Transgenic lines were: UAS-gcm ( F18A (one transgene) = weak-gcm ; M24A (two transgenes)= strong-gcm ) [16] ; gcm rA87 /CyO (weak hypomorph), gcm 34 /CyO,twi-LacZ (hypomorph), gcm 26 /CyO,twi-LacZ (null), Df(2L)132/CyO,twi-LacZ (null allele) [2] , [5] ; repo 3692 /TM3Ubx-lacZ [9] ; UAS–gcmFlag ; UAS-repo [11] ; UAS-dCBP and UAS-CBP FLAD [30] ; 2kb-gcm [12] ; nej [3] (dCBP null) [50] ; UAS-GFP , hs-gal4 , and sca-gal4 (BDSC). The gcm hypomorphic combinations shown in Supplementary Fig. 4k,l are: gcm rA87 /gcm 26 (weak), gcm 34 /gcm 34 (medium, same as columns 7,8 Fig. 7a ), gcm 34 /Df(2L)132 (strong, same as columns 5,6 Fig. 7a ). The medium UAS-gcm transgene in Supplementary Fig. 4m (and Fig. 7a gcm transgenes) was RS1 [31] . The repo-RFP line carries 4.3kb promoter of the repo gene fused with the RFP coding sequence. This fragment recapitulates the expression profile of the endogenous repo gene [34] . To compare the protein levels on Gcm mutagenesis, three lines were generated by targeted transgenesis into the ZH-attP-68E genomic site (III chromosome) [51] : UAS–gcmFlag , UAS–gcmFlag K>R and UAS–gcmFlag K>Q . IHC and in situ hybridization Overnight or staged embryos were dechorionated in bleach for 5 min, rinsed in water, fixed in 50% heptane/50% PEM-formaldehyde for 25 min and devitellinized in methanol/heptane for 1 min. The in situ hybridization was carried out using a probe DIG- gcm [1:100] [52] , [53] . For the immunolabelling, the embryos were rinsed in methanol, in phosphate-buffered saline (PBS) 0.3% Triton X-100, and incubated in blocking reagent (Roche) for 30 min at room temperature (RT). The embryos were incubated with primary antibody in blocking reagent overnight at 4 °C, washed in PBS 3 × 10 min at RT, incubated with secondary antibodies for 2 h at RT and washed 3 × 10 min at RT [5] . The embryos were mounted in Vectashield (Vector #H-1000) and analysed by conventional (Zeiss Axiophot) or confocal microscopy (SP5 Leica confocal microscope). Antibodies were as follows: mouse (m)-α-Repo (1:50) and rat (rt)-α-Elav (1:200) from DSHB; chicken (ck)-α-GFP (1:1,000); rabbit (rb)-α-RFP (1:500) and rb-α-Flag (Abcam); rb-α-GFP (1:500) (Molecular Probes); rb-α-β-gal (1:500, Cappel); rb-α-Eagle [1:500] [54] ; guinea pig-α-Deadpan (1:1,000, J. Skeath); rt-α-Ttk69 [1:1,000] [55] . Secondary antibodies were FITC-, Cy3-, Cy5-conjugated (1:400, Jackson). Cell counting Using Imaris Bitplane, the following parameters were followed: (1) three-dimensional masks were generated along the z-stacks of the embryonic ventral nerve cord (VNC) as regions of interest; (2) the number of cells was identified using the following parameters: select ‘Enable smooth’, surface area detail=0.5, select ‘Enable eliminate background’, diameter of largest sphere=5 μm, threshold=30, region growing estimated diameter=3, region grooving background subtraction=true, quality above 10, number of voxels above 10. The false negative is eliminated manually using Imaris tool on three-dimensional visualization of the VNC. Mean and s.e.m. were calculated for all genotypes and samples were subjected to t -test. Protein intensity measurement GcmFlag and GFP intensity measurements were done by ImageJ tool [20] . Masks were generated as region of interest for a defined area in the VNC of embryo the z-stack (10 μm), and the fluorescence intensities (pixel number) were measured and summed for all sections. The resulted intensities were subjected to t -test. qPCR analysis and mutagenesis Staged embryos were collected from the different genotypes. Total RNA was purified using Trizol (Invitrogen), reverse transcribed by SuperScript II and the qPCR was done with the Roche LightCycler480 and Sybr Green Master mix (Roche). Expression levels were automatically calculated (LightCycler480 Software, release 1.5.0) by calibration to gene-specific standard curves generated on input cDNAs [31] . Collected values were normalized to GFP messenger RNA amount, derived from four amplification reactions, each performed on four independent experiments. Primers are in Supplementary Table 1 . Cell culture and transfection assays Drosophila S2 cells were cultured in Schneider’s medium (Fisher Scientific). Cells (6 × 10 6 ) were cultured in 6-well plates 12 h before transfection. Each well was transfected with expression vectors: pActin-gcmFlag ( pAct-gcmFlag ) [21] , pActin-repo ( pAct-repo ) [11] , p Actin-dCBP ( pAct-dCBP ) [50] , pActin-lacZ ( pAct-lacZ ), pActin-gal4 ( pAct-gal4 ), pUAST-eGFP ( pUAS-GFP ), p6kb-gcm-gal4 , as indicated using 10 μl per 1 μg of DNA of Lipofectamine (Sigma). When required, pAct vector was added as carrier. Forty-eight hours post transfection, cells were lysed. Transfection efficiencies were normalized as specified in the legend to β-gal or GFP. Each experiment was performed at least three times. For drug treatments, 45 h post transfection, cells were treated 3 h with 20 μM of the proteasome inhibitor MG132 (Sigma), 30 μM of CBP/p300 inhibitor C646 (BioVision) or 30 μM Trichostatin (Sigma) cells. Immunoblot analysis Proteins were extracted from staged embryos from the specified genotypes [31] . A total of 30 μg of protein was separated by 8% SDS–PAGE gel, transferred onto nitrocellulose membrane and probed with primary antibodies diluted in 1 × PBS, 3% milk: m-α-Flag (1:5,000) (Sigma), ck-α-GFP (1:5,000) (Abcam), m-α-β-gal (1:1,000), m-α-Repo (1:2,000) (DSHB), rb-α-dCBP (1:5,000) (M. Mannervik). Signal was detected using the Pierce ECL western blotting substrate (Thermo Fisher Scientific) using HRP-conjugated secondary antibodies (1:5,000, Jackson). Chemiluminescence detection was performed according to manufacturer’s instructions (Amersham). Band quantifications used the ImageJ software. Gels submenu was used as indicated in ImageJ website. Results were compared using t -test. Full blots of each WB presented in the figures are presented in Supplementary Fig. 6 . Immunoprecipitation Transfected cells or staged embryos were lysed in the IP buffer (25 mM Tris–HCl pH 7.9, 10% (v/v) glycerol, 0.1% NP-40, 0.5 mM DTT, 5 mM MgCl2, 1 × proteinase inhibitor cocktail (Roche)). Protein lysates were immunoprecipitated with 100 μl protein G-Sepharose, for polyclonal dCBP antibody (Sigma), or A-Sepharose, for monoclonal Flag and Repo antibodies and ~5 μg of the different antibodies (as indicated). G/A-Sepharose protein–antibody–protein complexes were washed three times with the IP buffer comprising 0.5 M KCl and twice with buffer containing 100 mM KCl. After washing, protein-G-antibody-bound proteins were boiled in SDS sample buffer and analysed by WB. Acetylation was detected using rb-α-Ac-K (Cell Signaling #9441). Luciferase assay Double-stranded oligonucleotides covering the RBS of gcm promoter were synthesized. RBS 8 and RBS 9 were combined on the same oligonucleotide. Each oligonucleotide was designed with the WT RBS CAATTA and with a mutated RBS CAGTTA not bound by Repo [11] ( Supplementary Table 2 ). For each RBS, the double-stranded oligonucleotide was digested with 20 U of KpnI (NEB #R3142S) and 20 U of NheI (NEB #R3131S) in Cutsmart buffer (NEB #B7204S) for 1 h 30 min at 37 °C. The digested probe was cleaned using the PCR clean-up kit (MN #740609). A quantity of 1 μg of luciferase reporter plasmid pGL4.23[luc2/minP] ( pGL4.23 ) (Promega #E841A) was digested with KpnI and NheI as described previously, after 1 h 30 min at 37 °C, 20 U of CIP (Promega #M0290S) were added to the plasmid and incubated for 1 h at 37 °C. The plasmid was cleaned using the PCR clean-up kit (MN #740609). A quantity of 50 ng of digested luciferase plasmid was combined with the digested annealed probes (ratio plasmid:probe=1:6), 400 U of ligase (NEB #M0202S) and ligation buffer (NEB #B0202S) and incubated overnight at 18 °C. The ligated plasmids were then dialysed for 30 min on membrane filters (Millipore #VSWP02500) and amplified using the Plasmid DNA purification kit (MN #740410) according to manufacturer’s instructions. Transfections of S2 cells were carried out in 12-well plates using Effectene transfection reagent (Qiagen #301427). Cells were transfected with 0.5 μg pAct-lacZ , 0.5 μg pGL4.23 carrying the indicated RBS (or empty for the negative control), 0.5 μg pAct-repo or 0.5 μg pAct . Forty-eight hours after transfection, the cells were collected, washed once in cold PBS and resuspended in 100 μl of lysis buffer (25 mM Tris-phosphate pH7.8, 2 mM EDTA, 1 mM DTT, 10% glycerol, 1% Triton X-100). The suspensions were frozen/thawed four times in liquid nitrogen and centrifuged 30 min at 4 °C at 13,000 g . The activities of the Luciferase and the LacZ were measured in triplicate for each sample. For the LacZ measurement, 20 μl of lysate was mixed with 50 μl of βgal assay buffer (60 mM Na 2 PO 4 , 40 mM NaH 2 PO 4 , 10 mM KCl, 1 mM MgCl 2 , 50 mM β-mercaptoethanol) and 20 μl ONPG (4 mg ml −1 ) and incubated at 37 °C for 20 min. The reaction was stopped by adding 50 μl 1 M Na 2 CO 3 and the DO at 415 nm was measured. For the Luciferase activity, 10 μl of protein lysate was analysed on an opaque 96-well plate (Packard Instrument #6005290) with a Berthold Microluminat LB96P Luminometer by injecting 50 μl of luciferase buffer (20 mM Tris-phosphate pH 7.8, 1 mM MgCl 2 , 2.5 mM MgSO 4 , 0.1 mM EDTA, 0.5 mM ATP, 0.5 mM luciferin, 0.3 mM coenzyme A, 30 mM DTT). For both LacZ assay and Luciferase assay, the level of the background was estimated using lysate from S2 cells not transfected. The relative Luciferase levels were calculated as follows: the background was subtracted from each value, then the average of the technical triplicate were calculated. From there, the Luciferase activity of each sample was normalized to the LacZ activity (Luciferase activity/LacZ activity) to correct for transfection efficiency variability and the ratio (Luciferase with Repo/Luciferase without Repo) was calculated. For each RBS WT and mutant, biological triplicates were carried out. Repo chromatin IP The chromatin IP (ChIP) was performed according to standard protocols [56] , [57] with modification. A quantity of 100 mg of embryos w 1118 stage 11 was homogenized with a Dounce homogenizer in 1 × PBS, 0.4% formaldehyde and incubated 10 min at RT. Glycine was added to 0.2 M, the chromatin was incubated 10 min at RT and centrifuged 5 min at 500 g at 4 °C. The pellet was rinsed with cold PBS and resuspended in sonication buffer (50 mM HEPES pH8, 140 mM NaCl, 1 mM EDTA, 1% Triton X-100, 0.1% Na-deoxycholate, 0.25% SDS, 0.5 mM phenylmethanesulphonyl fluoride (PMSF), 1 × protease inhibitor complex) and incubated 5 min on ice. The lysate was sonicated 2 × 15 min (30 s on/30 s off) with a Diagenode water bath sonicator and centrifuged 15 min at 13,000 g at 4 °C. The supernatant was diluted 2.5 times in dilution buffer (15 mM Tris–HCl pH8, 150 mM NaCl, 1 mM EDTA, 1% Triton X-100, 0.1% SDS), 50 μg of diluted chromatin were used per ChIP. The chromatin solution was precleared 2 h at 4 °C with 40 μl of protein A Sepharose beads (Sigma #p3391) blocked with salmon sperm and BSA then centrifuged at 1,000 g for 5 min. The supernatant was incubated overnight at 4 °C with agitation with 5 μg of mouse anti-Repo antibody (DSHB #8D12) or with 5 μg of mouse IgG for the negative control; 40 μl of blocked protein-A Sepharose beads were added to the chromatin and incubated 1 h at 4 °C with agitation. The beads were pelleted 2 min at 500 g at 4 °C and washed twice 10 min with the following buffer: low-salt wash buffer (20 mM Tris pH8, 150 mM NaCl, 2 mM EDTA, 1% Triton X-100, 0.1% SDS), high-salt wash buffer (20 mM Tris pH8, 500 mM NaCl, 2 mM EDTA, 1% Triton X-100, 0.1% SDS), LiCl wash buffer (10mM Tris pH8, 1 mM EDTA, 0.25 M LiCl, 1% Na-deoxycholate, 1% NP-40) and TE buffer. The chromatin was eluted twice 15 min at RT with 250 μl elution buffer (100 mM NaHCO 3 , 1% SDS), 20 μl of NaCl 5M was added and the chromatin was incubated at 65 °C overnight, then 10 μg RNAse A was added and incubated for 1 h at 37 °C and 20 μg of proteinase K, 10 μl Tris–HCl pH6.8 2M and 10 μl EDTA 0.5M were added and incubated 1 h at 42 °C. The DNA was extracted with phenol/chloroform and resuspended in 20 μl water. A quantity of 5 ng of chromatin were used per qPCR using SYBR Green (Roche) in 10 μl with primers targeting each RBS of gcm promoter and primers designed in a region of gcm2 carrying no RBS for a negative control ( Supplementary Table 3 ). The enrichment was calculated for each RBS with the following formula: 2 (Ct_Chip_IgG−Ct_Chip_Repo) . Three biological replicates were done. Electrophoretic mobility shift assays hs-gal4>gcm synchronized embryos were submitted to 1-h heat-shock at 37 °C ((4–5 h) after egg laying) and raised to differentiate 6 h at 25 °C. Embryos were collected in Schneider’s medium, 3 mM EDTA and dissociated (Wheaton Dounce homogenizer). Cell suspensions were obtained on centrifugation (100 g , 5 min). Cells were washed with 1 × PBS and incubated 10 min at 4 °C in buffer A (10 mM HEPES–KOH pH 7.9, 1.5 mM MgCl 2 , 10 mM KCl, 0.5 mM DTT, 0.2 mM PMSF). After centrifugation of 10 s, the pellet was resuspended in buffer C (20 mM HEPES–KOH pH 7.9, 25% glycerol, 420 mM NaCl, 1.5 mM MgCl 2 , 0.2 mM EDTA, 0.5 mM DTT, 0.2 mM PMSF) for high salt extraction. Cellular debris were removed by centrifugation for 2 min at 4 °C and DNA binding proteins were stored at −80 °C. The profile of Repo was verified by WB analysis. Around 10 μg of nuclear extract was used in binding assays [12] . RBS 1 probe: 5′-TCTCATATCGTACAATTACCCAGTGGAGCG-3′. Mutagenesis of GcmFlag lysines GcmFlag sequence was mutated as follows: K120R, K124R, K128R and K179R (K>R mutations) or K120Q, K124Q, K128Q and K179Q (K>Q mutations) using pAct-gcmFlag [21] as template. For each mutant, three segments were synthesized separately (primers in Supplementary Table 4 ). For each segment, PCRs were done on 50 ng of pAct-gcmFlag using Expand High fidelity PCR system (Roche #11732641001) and the PCR programme: 94 °C 2 min, (94 °C 15 s, 50 °C 30 s, 72 °C 1 min 30 s) × 25 cycles and 72 °C 7 min. The segments were extracted from 1% agarose gel using Nucleospin PCR clean-up (MN #740609). The three segments were combined in equimolar concentration and a second round of PCR was performed with the primers ‘first segment K>R forward’ and ‘third segment K>R reverse’, using the Expand High fidelity PCR system with the following PCR programme: 94 °C 2 min, (94 °C 15 s, 45 °C 30 s, 72 °C 1 min 30 s) × 5 cycles, (94 °C 15 s, 55 °C 30 s, 72 °C 1 min 30 s) × 25 cycles and 72 °C 7 min. The PCR products gcmFlag K>R of around 1.8kb were gel extracted as above. The PCR products gcmFlag K>R and gcmFlag K>Q were digested with 20 U EcoR1-HF (NEB #R3101S) and 20 U Xba1 (NEB #R0145S) overnight at 37 °C in NEB buffer 2 (NEB #B7002S). Restriction enzymes were heat inactivated at 65 °C 20 min and the PCR product was cleaned with Nucleospin PCR clean-up. The plasmids pUAST and pAct were digested with EcoR1 and Xba1 as described previously and treated with CIP (NEB #M0290S) according to manufacturer’s instructions. The digested plasmids were purified using Nucleospin PCR clean-up. The ligations were carried out overnight at 18 °C with 50 ng of digested plasmids and 100 ng of digested PCR products gcmFlag K>R or gcmFlag K>Q using T4 DNA ligase (NEB #M0202S) according to the manufacturer’s instruction. The ligation products were dialyzed on 0.025 MF mixed cellulose ester membrane (Millipore #VSWP02500), electroporated into DH5α competent cells and isolated using NucleoSpin Plasmid kit. The integrity of the sequences of gcmFlag K>R and gcmFlag K>Q was assessed by Sanger sequencing using the primers: pUAST_F (5′-taaccagcaaccaagtaaatc-3′) and pUAST_R (5′-ctcccattcatcagttccat-3′), the primers first segment K>R Forward and third segment reverse for the pPAC5C. Mutated GcmFlag stability and activity S2 cells were transfected with 1 μg of one of the following expression vectors: pUAS-gcmFlag K>R , pUAS-gcmFlag K>Q , pUAS-gcmFlag and with 1 μg of pUAS-lacZ , 1 μg of pAct-gal4 and 1 μg of 4.3kb -repo-GFP [14] using the Effectene transfection reagent (Qiagen). Forty-eight hours post transfection, the cells were collected, lysed in 25 mM Tris–HCl pH 7.9, 10% glycerol, 0.1% NP-40, 0.5 mM DTT, 5 mM MgCl 2 , 1 × protease inhibitor (Roche #11836153001), frozen–thawed four times in liquid nitrogen and centrifuged at 13,000 g 10 min at 4 °C. The supernatant was collected, its concentration was measured using nanodrop and immunoblots were performed with 50 μg of protein of each sample, primary antibody targeting Flag (1:5,000) (Sigma), GFP (1:5,000) (Abcam) and β-gal (1:1,000) and HRP-conjugated secondary antibodies, as described previously. Each transfection was performed at least three times, the results were compared using t -test. Mutated GcmFlag stability and activity in presence of CBP Drosophila S2 cells were transfected with 1 μg of one of the following expression vectors: pAct-gcmFlag K>R , pAct-gcmFlag K>Q, pAct-gcmFlag and with 1 μg of pAct-lacZ , 1 μg of 4.3kb -repo-GFP [14] and in CBP+ samples 1 μg of p Act-dCBP [50] using the Effectene transfection reagent (Qiagen #301427). When required, the pAct vector was added as carrier. Forty-eight hours post transfection, GFP-positive cells were counted using ImageJ tools, then the cells were collected, lysed in 25 mM Tris–HCl pH 7.9, 10% glycerol, 0.1% NP-40, 0.5 mM DTT, 5 mM MgCl 2 , 1 × protease inhibitor (Roche #11836153001), frozen–thawed four times in liquid nitrogen and centrifuged at 13,000 g 10 min at 4 °C. The supernatant was collected, its concentration was measured using nanodrop and immunoblots were performed with 50 μg of protein of each sample, primary antibody targeting Flag (1:5,000) (Sigma), GFP (1:5,000) (Abcam) and β-gal (1:1,000) and HRP-conjugated secondary antibodies, as described previously. Each transfection was performed at least three times and the results were compared using t -test. In vitro acetylation and mass spectrometry analysis The CBP HAT domain, GST-dCBP 1675–2510, was produced in BL21 cells, purified on glutathione sepharose beads [58] and eluted with thrombin. Similarly, sequences encoding the 115 first amino acids (Gcm115) and 202 first amino acids of Gcm (Gcm202) were cloned in pGex4T3 vector [4] produced in BL21 cells and bound to glutathione sepharose beads. The in vitro acetylation was carried out directly on the beads with 1 μg or 4 μg purified CBP in 5% glycerol, 50 mM NaCl, 50 mM Tris pH8, 0.1 mM EDTA, 10 mM Na-butyrate, 1 mM DTT, 1 × protease inhibitor complex Roche #04693116001), 30 μM acetyl-coenzyme A for 1 h at 30 °C [59] . The beads carrying Gcm–DBD 115 aa or Gcm–DBD 202 aa were washed twice with PBS and eluted with 1 U of thrombin overnight at RT. The eluted proteins were analysed by WB targeting acetylated lysine. Acetylated Gcm202 was analysed by mass spectrometry to identify the acetylated lysines. The protein band was excised from a 15% SDS–PAGE coloured by Coomassie blue, digested with chymotrypsin (Promega) or ArgC (Roche) and analysed with a Hybrid Ion Trap-Orbitrap Mass Spectrometer coupled with a nanoRSLC system (ThermoScientific). The protocol is detailed in Supplementary Methods . How to cite this article : Flici, H. et al . Interlocked loops trigger lineage specification and stable fates in the Drosophila nervous system. Nat. Commun. 5:4484 doi: 10.1038/ncomms5484 (2014).